TheSpirodela polyrhizagenome reveals insights into its neotenous reduction fast growth and aquatic lifestyle The subfamily of the Lemnoideae belongs to a different order than other monocotyledonous species that have been sequenced and comprises aquatic plants that grow rapidly on the water surface. Here we select Spirodela polyrhiza for whole-genome sequencing. We show that Spirodela has a genome with no signs of recent retrotranspositions but signatures of two ancient whole-genome duplications, possibly 95 million years ago (mya), older than those in Arabidopsis and rice. Its genome has only 19,623 predicted protein-coding genes, which is 28% less than the dicotyledonous Arabidopsis thaliana and 50% less than monocotyledonous rice. We propose that at least in part, the neotenous reduction of these aquatic plants is based on readjusted copy numbers of promoters and repressors of the juvenile-to-adult transition. The Spirodela genome, along with its unique biology and physiology, will stimulate new insights into environmental adaptation, ecology, evolution and plant development, and will be instrumental for future bioenergy applications. L emnoideae , commonly known as duckweeds, are the smallest, fastest growing and morphologically simplest of flowering plants [1] . The plant body is organized as a thalloid or ‘frond’ lacking a stem and in more derived species even roots ( Fig. 1 ). Based on fossil records, the peculiar plant body architecture of this subfamily evolved by neotenous reduction from an Araceae ancestor and it has been interpreted botanically as juvenile or embryonic tissue [2] . The reduction and simplification of the plant body progresses within the Lemnoideae from ancient species like Spirodela towards more derived species like Wolffia. Although reduced flowers are observed in duckweeds, they usually reproduce by vegetative daughter fronds initiated from the mother frond ( Supplementary Fig. 1 ). Doubling time of the fastest growing duckweeds under optimal growth conditions is <30 h, nearly twice as fast as other ‘fast-growing’ flowering plants and more than double that of conventional crops (more under Supplementary Note 1 ). They are easy to grow and have negligible lignin and high energy content in the form of easily fermentable starch (40–70% of biomass). Duckweeds have been used for the removal of high levels of contaminants from wastewater [3] and for the production of recombinant proteins for pharmaceutical applications [4] , [5] and high-impact biofuel feedstock that does not compete for land in food production [6] . From a taxonomic point of view, genomic efforts have largely focused on the taxa of the Commelinid monocots such as the grasses from Poales and Musa acuminata , the wild-type diploid progenitor of banana, from Zingiberales ( Fig. 1 ). 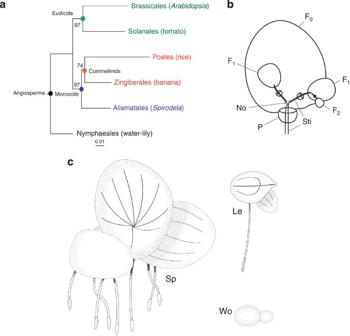Figure 1:Systematics and biology of theLemnoideae. Duckweeds belong to the orderAlismatalesand theAraceaefamily, an early branch-off from the monocotyledonous crown ancestor. In agreement with previous classifications70, (a) shows a phylogenetic tree of plastid-rbcL (ribulose-1, 5-bisphosphate carboxylase large-subunit) genes of two dicots—Arabidopsis thaliana(Brassicales, NC_000932.1) and tomato (Solanales, NC_007898.2); three monocotsSpirodela polyrhiza(Alismatales, NC_015891.1), rice (Poales, NC_001320.1) and banana (Zingiberales, EU017045.1), and water-lily as an outgroup (Nuphar advena,Nymphaeales, NC_008788). (b) shows a ventral view of Spirodela, illustrating schematically the clonal, vegetative propagation of duckweeds (redrawn and simplified from Landolt26). Daughter fronds (F1) originate from the vegetative node (No), from the mother frond F0 and remain attached to it by the stipule (Sti), which eventually breaks off, thereby releasing a new plant cluster. Daughter fronds may already initiate new fronds (F2) themselves before full maturity. Roots are attached at the prophyllum (P). (c) illustrates the progressive reduction from a leaf-like body with several veins and unbranched roots to a thallus-like morphology in theLemnoideae, redrawn after historical illustrations ‘Das Pflanzenreich’ fromwww.biolib.de; Sp:Spirodela polyrhiza, Le:Lemna minor, Wo:Wolffia arrhiza. Figure 1: Systematics and biology of the Lemnoideae . Duckweeds belong to the order Alismatales and the Araceae family, an early branch-off from the monocotyledonous crown ancestor. In agreement with previous classifications [70] , ( a ) shows a phylogenetic tree of plastid-rbcL (ribulose-1, 5-bisphosphate carboxylase large-subunit) genes of two dicots— Arabidopsis thaliana ( Brassicales , NC_000932.1) and tomato ( Solanales , NC_007898.2); three monocots Spirodela polyrhiza ( Alismatales , NC_015891.1), rice ( Poales , NC_001320.1) and banana ( Zingiberales , EU017045.1), and water-lily as an outgroup ( Nuphar advena , Nymphaeales , NC_008788). ( b ) shows a ventral view of Spirodela, illustrating schematically the clonal, vegetative propagation of duckweeds (redrawn and simplified from Landolt [26] ). Daughter fronds (F1) originate from the vegetative node (No), from the mother frond F0 and remain attached to it by the stipule (Sti), which eventually breaks off, thereby releasing a new plant cluster. Daughter fronds may already initiate new fronds (F2) themselves before full maturity. Roots are attached at the prophyllum (P). ( c ) illustrates the progressive reduction from a leaf-like body with several veins and unbranched roots to a thallus-like morphology in the Lemnoideae , redrawn after historical illustrations ‘Das Pflanzenreich’ from www.biolib.de ; Sp: Spirodela polyrhiza , Le: Lemna minor , Wo: Wolffia arrhiza . Full size image Here we describe the genome and transcriptome of Greater Duckweed, Spirodela polyrhiza , representing the smallest monocot genome to date with a size of 158 Mb, which is similar to the plant model genome of Arabidopsis thaliana . Spirodela represents a basal monocotyledonous species from the Alismatales and will be an invaluable genomic resource to study the history of the monocotyledonous lineage. Sequence assembly Genome sizes in the five Lemnoideae genera span an order of magnitude from 158 Mb in Spirodela polyrhiza to 1,881 Mb in Wolffia arrhiza [7] . Owing to its small size and basal position in the Lemnoideae we sequenced the Spirodela polyrhiza strain 7498 by whole-genome shotgun sequencing using ~20 × single end, ~1 × pair-end Roche/454 next-generation sequencing and ~1 × pair-end Sanger sequencing as described under Methods ( Supplementary Table 1 ). Although next-generation sequencing has been used to reduce the cost of sequencing genomes, short-read technologies have been insufficient to assemble chromosome-size molecules with megabase (Mb) genomes, especially for Spirodela, which does not have synteny with other fully sequenced genomes. Therefore, the read-length threshold of Roche/454 with a depth of 21 × in combination with long paired-reads from BACs and fosmids appeared to be a significant improvement in the balance of cost and genome sequence quality for new evolutionary references. Of the 158-Mb genome, as measured by flow cytometry ( Supplementary Fig. 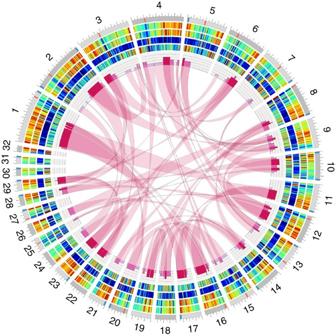Figure 2: Characteristics of the Spirodela genome. The outer circle shows the 32 pseudomolecules of the Spirodela genome assembly, tick scaling is 500 kb and blue and red bars depict position of telomeric and centromeric clusters. Heatmap tracks illustrate from outer to inner circle GC content, gene, repeat and GAGA-repeat densities. Colour map ranges are 30–50%, 0–30%, 0–70% and 0–1.5%, respectively. GC and gene content are positively, repeat and gene densities negatively correlated, whereas GAGA-repeats are present both in gene- and repeat-rich regions. The genome contains two rounds of ancient genome duplications. For each genomic segment, the copy number of paralogous regions is shown as bar chart in the innermost circle, duplication history is illustrated by red ribbons. 2 ), 90% was assembled into contigs, 97% of the contigs assembled in 252 scaffolds and 94.1% of them in the top 50 largest scaffolds ( Supplementary Table 2 ). To align the scaffolds with chromosomes, we constructed a Spirodela genomic library of bacterial artificial chromosomes (BACs) that was subjected to DNA fingerprinting, resulting in a physical map (Methods). BAC end sequences (BES) were used to align the assembled sequences with the physical map, providing us with proof of an accurate assembly of DNA sequences. We also used BACs that were aligned to the assembly with their sequenced ends to derive their entire sequence from the assembled sequences and used this information to select those that were low in repeat sequences for fluorescence in situ hybridization (FISH). Scaffolds were joined into 32 pseudomolecules, using the DNA fingerprinted physical map with anchored sequenced tagged sites (BESs), and one pseudomolecule labelled ‘0’ with all unanchored scaffolds ( Fig. 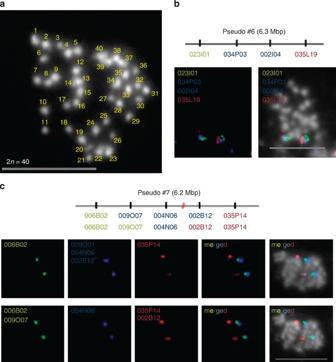Figure 3: Cytogenetics by FISH. (a) Metaphase spread indicating a chromosome number of 2n=40 forSpirodela polyrhiza7498. (b) Validation of BAC positions on a single chromosome pair by anchoring pseudo#6 ofSpirodela polyrhizavia multicolour FISH. (c) The chimeric pseudo#7 was revealed by reprobing BACs with different fluorescence color schemes. Scale bars, 10 um. 2 ); ( Supplementary Table 3 ). Gaps in sequences like centromeres amounted to 10.7% of the genome and remained in unnamed bases (Ns). Figure 2: Characteristics of the Spirodela genome. The outer circle shows the 32 pseudomolecules of the Spirodela genome assembly, tick scaling is 500 kb and blue and red bars depict position of telomeric and centromeric clusters. Heatmap tracks illustrate from outer to inner circle GC content, gene, repeat and GAGA-repeat densities. Colour map ranges are 30–50%, 0–30%, 0–70% and 0–1.5%, respectively. GC and gene content are positively, repeat and gene densities negatively correlated, whereas GAGA-repeats are present both in gene- and repeat-rich regions. The genome contains two rounds of ancient genome duplications. For each genomic segment, the copy number of paralogous regions is shown as bar chart in the innermost circle, duplication history is illustrated by red ribbons. Full size image To examine how the 32 pseudomolecules relate to the 20 chromosomes of the haploid genome of Spirodela polyrhiza , we applied a cytogenetic analysis as described under Methods. FISH data supported the coherence of the 32 BAC-based pseudomolecules in distinct chromosome pairs ( Fig. 3 ). In two cases (pseudo #7 and #21) individual BACs were located on chromosomes other than the remaining contig. For instance, 002B12 and 035P14 labelled another chromosome than the other three BACs of pseudo #7. Thus, these two pseudomolecules were chimeric and each of the two arms had to be separated and joined to another arm to form one of the 20 chromosomes. Chimerism of pseudomolecules could be due to the short reads of the ‘454’ sequencing–platform and repeat-dense regions of the chromosomes. Although future work will have to convert pseudomolecules into chromosomes, the current analysis of the gene content and order remained unaffected. Figure 3: Cytogenetics by FISH. ( a ) Metaphase spread indicating a chromosome number of 2 n =40 for Spirodela polyrhiza 7498. ( b ) Validation of BAC positions on a single chromosome pair by anchoring pseudo#6 of Spirodela polyrhiza via multicolour FISH. ( c ) The chimeric pseudo#7 was revealed by reprobing BACs with different fluorescence color schemes. Scale bars, 10 um. Full size image To confirm that no other chimerism underlies the overall assembly quality and completeness, we localized telomeric repeats in the pseudomolecules. In higher plants, telomeres are characterized by tandem repeats of the conserved heptamer sequence TTTAGGG. Clusters of telomeric repeats were exclusively identified at the ends of the pseudomolecules, supporting the assumption that there were no hybrids of chromosomal arms ( Supplementary Fig. 3 ). Confirmation of the accuracy of sequence assembly was also possible with the distribution of repeat elements in the pseudomolecules described further below. As an additional quantitative assessment of the completeness of the sequence assembly the Spirodela pseudomolecules were scanned for their content of ESTs, BES and 454 reads via masking ( Supplementary Fig. 4 , assembly checker method). Three different-sized batches of randomly sampled 454 reads with 1, 2 and 5 × genome coverage, corresponding to Lander-Waterman statistics of 63, 87 and 99%, served as calibration sets with known genomic coverage. The Spirodela assembly contained 80% of the 1 × read test set and 90% of the EST and BES test sets. The content values for ESTs and BES were almost identical to the 5 × read set, which should represent the whole sequence amount. Overall the assembly completeness could be verified with the described new masking method to be at least 90% for genic sequences and ≥80% for the rest, which is in the same range as the values given in Supplementary Tables 4 and 5 (95.7% for ESTs, 83% for AraCyc genes). To further ensure the quality of sequence assembly, we randomly selected 24 fosmids for conventional sequencing that were then aligned with the assembled 454 sequences and found that the sequencing error rates were 8 in 10,000, providing 98.22% accuracy ( Supplementary Table 6 ). Repeat elements The major sources of repeat elements in the genome are transposons and variable number tandem repeats (VNTRs). 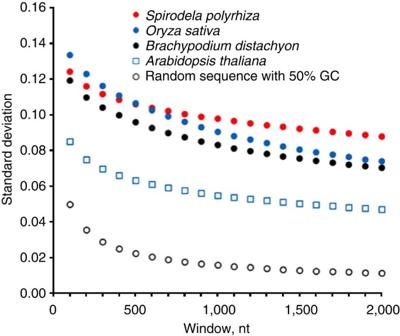Figure 6: Comparison of genome compositional heterogeneity in several plants. Standard deviation (s.d.) of GC content within a sequence fragment (window) is shown as a function of the window size for several plants and a random nucleotide sequence. The level of composition heterogeneity of genomic sequence is measured by s.d. of GC content defined in fragments of fixed length sampled along the genome. Other sources like high copy number genes (for example, rRNA genes) and different degrees of duplications (polyploidy, segmental duplications and tandem genes) usually contribute only to far lesser extent to total repeat sequences. To identify common and special features of the Spirodela genome the repeat data were put into a comparative context with the similar-sized Arabidopsis thaliana (At) (tigr 8 version) [8] and three to four monocot genomes of different sizes, Brachpodium distachyon (Bd) [9] , Oryza sativa (rice) (Os) [10] , Sorghum bicolour (Sb) [11] and Zea mays (maize) (Zm) [12] ( Supplementary Fig. 5 ). Comparing the 16mer frequency of Spirodela with other plant genomes shows that the kmer curve of Spirodela follows a similar trend as the equally sized Arabidopsis genome. In both genomes kmers occurring ≥10 times are only found in ~3–4% of the sequence. In the larger monocot genomes, there is a continuous rise towards increase of genome size with kmers repeated ≥10 times starting from 12% in Brachypodium up to 63% in sorghum. A homology search with de novo full-length long terminal repeat (LTR)-retrotransposons traces 13% of the Spirodela genome as LTR-retrotransposon-derived, which is perfectly in line with its small genome size ( Fig. 4 ). A surprising result was the ratio of gypsy/copia LTR-retrotransposons of 3.5 in Spirodela, next to sorghum the second highest among the five genomes ( Table 1 ). An annotation attempt with RepeatMasker against mips-REdat_v9.3 (ref. 13 ) gave an additional 2.5% of retroelements and 0.23% of DNA transposons. A closer inspection revealed that the DNA transposon hits were only based on small stretches of simple sequence repeats, which occurred within the template transposon sequence. The same and related problems were true for the additional retroelement hits from other species. Owing to their largely unspecific nature all transposon hits from non-Spirodela template sequences were removed from the final annotation. 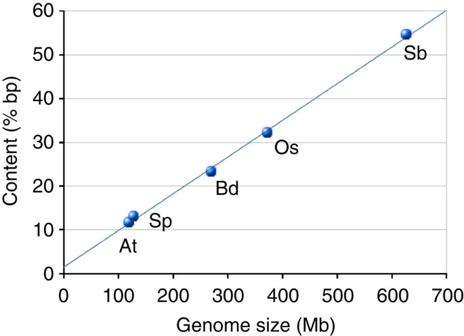The observed lack of transposon similarity confirmed the large evolutionary distance between Spirodela and sequenced monocot genomes. Figure 4: Linear dependency between genome size and LTR retrotransposon content for small-sized (<<1 Gb) plant genomes. Percentage of repetitive DNA is plotted against the genome size of different plant genomes, At for Arabidopsis, Sp for Spirodela, Bd for Brachypodium, Os for rice and Sb for sorghum. Figure 4: Linear dependency between genome size and LTR retrotransposon content for small-sized (<<1 Gb) plant genomes. Percentage of repetitive DNA is plotted against the genome size of different plant genomes, At for Arabidopsis, Sp for Spirodela, Bd for Brachypodium, Os for rice and Sb for sorghum. Full size image Table 1 Repeat composition of Spirodela compared with other plant genomes. Full size table The percentage of tandem repeats (VTNRs) found in genome assemblies is relatively independent of genome size and ranged usually between ~2 to 3% ( Table 1 ). The higher satellite repeat content of sorghum can be explained by its fully sequenced centromeres for three chromosomes. Spirodela has an exceptionally high proportion of microsatellite tandem repeats, 50% versus 3 to 6% in four reference genomes ( Fig. 5 ). This amplification even influences the absolute amounts of microsatellite repeats, as Spirodela tops the list with 1 Mb followed by the much larger sorghum genome with 0.9 Mb ( Fig. 5b ). A detailed breakdown of microsatellite repeats into the different monomer sizes shows that one of the four possible dinucleotide repeats, namely ‘GAGA’, is responsible for the noticeable increased numbers of microsatellite repeats ( Supplementary Fig. 6 ). 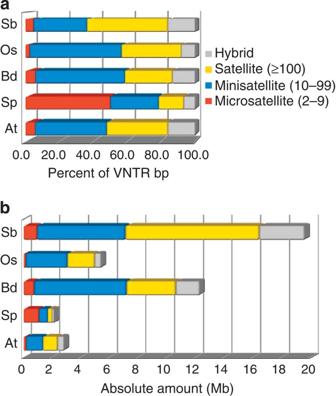Owing to their high repetition, they severely impeded elongation during sequence assembly and were prevalently found at one or both ends of a pseudomolecule together with very high 16mer frequencies, especially often in the unplaced contigs of pseudo #0. Figure 5: Composition of tandem repeat. (a) The percentage of tandem repeats in different plant genomes were broken down into satellite (yellow), minisatellite (blue), microsatellite (red) and composite satellite (grey) sequences. (b) The same comparison was made with respect to the absolute amount in Mb. Genomes were ordered according to size, with the lowest at the bottom, At for Arabidopsis, Sp for Spirodela, Bd for Brachypodium, Os for rice and Sb for sorghum. Figure 5: Composition of tandem repeat. ( a ) The percentage of tandem repeats in different plant genomes were broken down into satellite (yellow), minisatellite (blue), microsatellite (red) and composite satellite (grey) sequences. ( b ) The same comparison was made with respect to the absolute amount in Mb. Genomes were ordered according to size, with the lowest at the bottom, At for Arabidopsis, Sp for Spirodela, Bd for Brachypodium, Os for rice and Sb for sorghum. Full size image Although Spirodela harbours almost the same amount of full-length LTR retrotransposons as the similar-sized Arabidopsis genome, the insertions are distinctly older (average 4.6 versus 2.0 mya) and very young elements have not been found. The age pattern of LTR-retrotransposon insertions in Spirodela shows distinct differences to other genomes, even to Arabidopsis. The Spirodela insertions are spread out over a longer time period, leading to higher average and median age values. The complete absence of very young full-length LTR-retrotransposons should be treated with caution, since it could also be an artefact of the ‘454’ sequencing platform, where identical sequence stretches tend to collapse. Still, the atypical age distribution suggests an ‘ancient’ genome state without much recent transposon activity in combination with small removal rates. The common picture in plant genomes of younger copia and older gypsy LTR-retrotransposons is weakly visible in Spirodela ( Supplementary Fig. 7 ). The small genome size and atypical LTR age distribution of Spirodela suggested a tight control of transposon activity during recent evolutionary times. Both features might well be connected to the continuous clonal propagation of Spirodela. Transposon transcription is usually activated during seed development [14] and full-length LTR-retrotransposon elements are often removed by meiotic unequal crossing over between solo LTRs [15] , two processes that are limited by the propensity of Spirodela to an asexual lifestyle. Also, in small genomes undergoing genome size reduction, transposition potentially could negatively impact gene activity, possibly requiring tighter regulation. Gene number and transcriptome After the determination of repeat elements in the Spirodela genome these sequences could be filtered out to make the prediction pipeline for the gene content and their order in the 32 pseudomolecules more specific. We could identify 19,623 protein-coding genes in Spirodela (Methods), 28% less than Arabidopsis (27,416) and 50% less than rice (39,049) ( Table 2 ). Sources of other genomes and normalization of data sets are described under Supplementary Discussion . 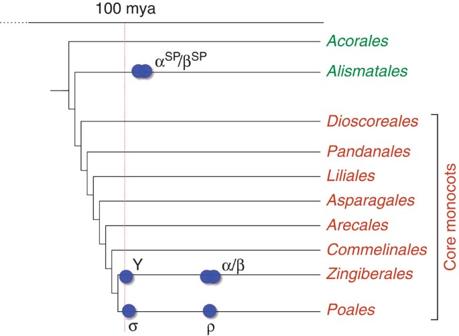Figure 7: Phylogeny of monocotyledonous orders. The dendrogram is a simplified version redrawn from ref.18. Core monocots are shown in brown, known WGDs are shown as blue circles. The Spirodela gene models were supported by 379,502 EST sequences assembled from transcriptome libraries generated from various diurnal time course and stress conditions ( Supplementary Table 7 ). An unusual aspect of the gene content in the Spirodela genome is the local variability in GC composition, which exceeds variability observed in other plant genomes ( Fig. 6 ). Also, the differences between exon and intron GC content vary significantly between genes ( Supplementary Fig. 8 ). Still, the new ab initio algorithm was able to predict in a single run 19,327 genes, the number close to the final number of genes in annotation. The accuracy of the new algorithm was shown to be sufficiently high by assessment on a test set generated from mapping the transcripts and high-quality proteins (Sn/Sp of exact prediction of internal exons: 87.2%/74.5%). Mean exon and coding sequence sizes were similar in all five genomes. However, Spirodela shared with banana significantly larger gene sizes, which apparently resulted from longer introns. Composition heterogeneity of genomic sequence can be measured by s.d. of GC in fragments sampled along the genome. At fragment length 2,000 nt, the s.d. of GC content in Arabidopsis thaliana is five times higher (5 × ) than in a random sequence, whereas in Spirodela polyrhiza it was observed to be 9 × , thus evident of much higher composition heterogeneity than in Arabidopsis thaliana and even higher than in rice (8 × ), which is notoriously difficult for the analysis of statistical patterns related to protein-coding regions ( Supplementary Fig. 9 ). Table 2 Gene characteristics. This table shows the statistics of gene features for three monocotyledonous species (spirodela, rice and banana) and two dicotylodonous species (tomato and arabidopsis). Full size table Figure 6: Comparison of genome compositional heterogeneity in several plants. Standard deviation (s.d.) of GC content within a sequence fragment (window) is shown as a function of the window size for several plants and a random nucleotide sequence. The level of composition heterogeneity of genomic sequence is measured by s.d. of GC content defined in fragments of fixed length sampled along the genome. Full size image Still, several lines of evidence supported the considerably lower gene number in Spirodela compared with other higher plant species. First, three independent gene prediction pipelines—the one described above, a self-training version of genemark and an approach using homology and transcriptome data—consistently predicted a gene number below 20,000 genes. Second, we observed a similar coverage of the AraCyc pathway genes [16] between monocotyledonous species: 87, 86 and 83% of the AraCyc genes were represented by a homologue (≥40% sequence identity, ≥70% alignment coverage) in the annotations of rice, banana and Spirodela, respectively ( Supplementary Table 5 ). In comparison to dicots, increased GC contents were observed in monocotyledonous coding sequences, mainly due to a mutational bias of G and C in the third codon position. Spirodela protein-coding sequences exhibited a pronounced GC3 bias ( Supplementary Fig. 9 ), which was the highest amongst currently sequenced monocot genomes ( Fig. 6 ). Elevated GC3 contents were found in Spirodela specific genes as well as genes shared with monocots and dicots and thus seemed to be a general feature of Spirodela-coding sequences ( Supplementary Fig. 10 ). In contrast to the reported distinct bimodal distributions in rice and maize, Arabidopsis genes showed a sharp unimodal distribution. Broader distributions resulting from a composite of genes with low and high GC3 content were observed both for banana and Spirodela genes ( Supplementary Fig. 9 ), suggesting that the distinct multimodal patterns evolved specifically, whereas high GC3 biases might have evolved independently and several times in the monocotyledonous lineage. 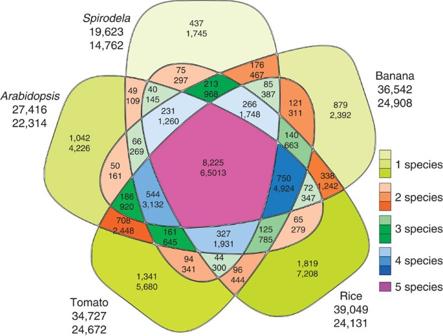Figure 8: OrthoMCL analysis of gene families. The Venn diagram illustrates shared and distinct cluster classes from an orthoMCL analysis of the plant proteomes ofArabidopsis thaliana,Solanum lycopersicum,Spirodela polyrhiza,Musa acuminataandOryza sativa spp. indica. Non-redundant data sets were used in the analysis. Numbers below each species name show number of all genes in species set and number of clustered genes, respectively. For each division in the Venn diagram, the top line shows the number of orthoMCL clusters and the bottom line the number of total genes in these clusters. The different cluster classes are colour-coded by the number of species containing genes for the respective class. Divisions for each class are shaded according to their abundance in their class with darker shades indicate larger contributions of the particular division. Gene clusters and miRNAs Spirodela appeared to have a significantly lower number of tandem gene clusters (948) than rice (2,602), tomato (2,340) and Arabidopsis (1,938); however, surprisingly close to banana (1,048), which had ~1.9 times the gene number of Spirodela ( Supplementary Table 8 ). Interestingly, genome sequences of the latter two genomes are largely based on assemblies of next-generation sequencing technologies and some very closely related tandem genes may have collapsed in the assembly of short reads. However, considering the proportion of tandem genes relative to all genes, Spirodela does not deviate so much from other species (15.6% versus 19–21%), as banana does (7%). Therefore, the observed lower number of tandem genes can only partially compensate for the lower gene count in Spirodela. 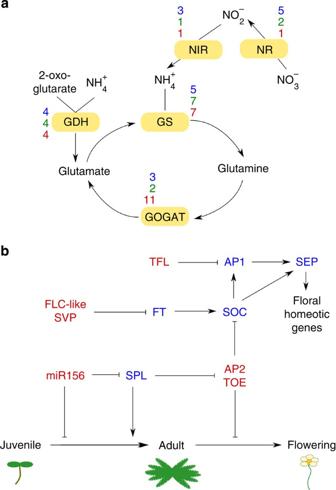Figure 9: Spirodela characteristic pathways. (a) A schematic diagram of nitrogen assimilation in higher plants is illustrated. Spirodela shows a high overrepresentation of enzymes of the GS/GOGAT cycle, the major module for ammonia assimilation and consistent with the high ability of Spirodela to remove ammonia from sewage and wastewaters. Copy numbers for each gene are shown in red for Spirodela, blue for rice and green for Arabidopsis. (b) A highly simplified scheme of the regulatory network of the juvenile-to-adult phase transition in Arabidopsis is illustrated. Most genes have several, functionally similar paralogs and are only shown for simplicity reasons by one gene symbol. For example, APETALA1, CAULIFLOWER and FRUITFUL are close paralogs promoting the onset of an inflorescence meristem but are represented only by one gene symbol, AP1. Gene groups having either similar copy numbers or being overrepresented in Spirodela are shown in red; those that have significantly reduced numbers are shown in blue. A total of 413 miRNA loci comprising 93 families were identified in the Spirodela genome assembly by sequence similarity and structural features as described under Methods ( Supplementary Table 9 ). Gene distribution along chromosomes The annotation of both repeat elements and genes allows us to make a graphic representation of gene and repeat densities along the chromosomes (Methods). The heat map of the Spirodela pseudomolecules follows the known pattern of anti-correlation between gene and LTR-retrotransposon share of plant genomes ( Supplementary Fig. 11 ). LTRs were largely absent from gene-rich regions but accumulate in gene-poor regions. There is a perfect correlation between prominent retrotransposon/kmer peaks and known centromeric locations in many other plant genomes (for example, sorghum, Brachypodium, rice, cotton, tomato and Arabidopsis). Here, based on high LTR-retrotransposon (>80–90%) content together with high kmer values, the constrictions are to be seen as the most likely positions of the centromeres. The whole length of pseudomolecule #2 is detailed in Supplementary Fig. 12 . Organelle insertions A total of 1,385 chloroplast DNA fragment insertions covering 240,242 bp (0.15%) of the nuclear genome were identified. In all, 1,320 insertions detected were shorter than 500 bp, with 34 between 0.5 and 1 kb, 21 between 1 and 2 kb, and only 10 exceeding 2 kb with the largest being 5,197 bp ( Supplementary Table 10 ). A total of 1,589 mtDNA insertions into the nuclear genome covering 207,711 bp (0.13%) had been detected. Similar to the findings for the chloroplast insertions, 1,554 were <500 bp in length, with 31 between 0.5 and 1 kb, 3 between 1 and 2 kb, and 1 exceeding 2 kb (2,185 bp) ( Supplementary Table 11 ). Genome evolution We determined the syntenic relations between rice and Spirodela as described under Methods. The dot plot suggested a quota for the syntenic relation of 2:4 for rice and Spirodela duplicated segments, respectively ( Supplementary Fig. 13 ), indicating that the well-known ρ-WGD in grasses and the αSP/βSP-WGDs in Spirodela occurred independently of each other. The reported σ-duplication in grasses predating ρ had recently been placed after the split of the Zingiberales and Poales [17] . This study also reported an additional γ-WGD that was specific to the Zingiberales and hence had occurred after the split of the Alismatales and the core monocots. The Alismatales —together with the Acorales— represent the most ancient monocotyledonous clade that diverged from the core monocots, which included for example the Commelinids , Asparagales and Liliales , ~130 mya (ref. 18 ). This placed the αSP/βSP-WGDs of Spirodela in the Alismatales branch ( Fig. 7 ). Figure 7: Phylogeny of monocotyledonous orders. The dendrogram is a simplified version redrawn from ref. 18 . Core monocots are shown in brown, known WGDs are shown as blue circles. Full size image Copy numbers of duplicated chromosomal segments provided further support for two rounds of WGDs in Spirodela ( Supplementary Fig. 14 ). For about one third of the genome, no duplicated counterpart was observed. However, segments with copy numbers of four comprised approximately a quarter of the available genome sequence and were the second largest copy number class, followed by segments with three and two copies in the genome. Syntenic conservation between segmental blocks was significantly lower compared with those reported for grasses. Although syntenic regions between sorghum and rice contained on average 58% of the genes in collinear blocks [11] , duplications in Spirodela showed a sparse conservation with a mean of 11.3% of syntenic paralogous pairs in collinear order ( Supplementary Table 12 ). This number might be an underestimate because global gene-based alignments between two blocks might miss small inversions or local translocations. Nevertheless, the reduced number was consistent with the older age of the presumed WGDs and a continuous loss of duplicated genes [19] . Synonymous substitution rates showed a unimodal distribution, indicating that both WGDs occurred within a short period of time ( Supplementary Fig. 15 ) and that they could not be separated by their divergence times. We therefore refer to the WGDs in Spirodela as αSP/βSP. There was a distinct shift in the mean peak K s values for GC3-high (mean ~0.85) and GC3-low (mean ~1.23) gene pairs. In this study and in agreement with other reports [20] , we used the GC3-low paralogous pairs to estimate the occurrence of both WGDs at ~95 mya, which was older than the previously reported ρ-WGD in grasses and the γ-WGD in the Zingiberales. Syntenic conservation of collinear gene pairs between rice and Spirodela was slightly higher than those of the αSP/βSP-WGDs, with a mean of 15% of co-orthologous pairs in the chromosomal segments showing conserved order. In total, the segments spanned 20,451 loci in rice and 11,479 in Spirodela, with 4,275 and 3,710 non-redundant collinear genes, respectively. Syntenic gene pairs between rice and Spirodela showed a pronounced bimodal distribution that was clearly caused by the superimposition of two unimodal distributions of GC3-high and GC3-low gene pairs ( Supplementary Fig. 16 ). Following this rationale, we determined a mean peak K s of ~1.7 for the GC3-low distribution translating into a divergence time of ~130 mya. This estimate closely agrees with the divergence of the Alismatales and the core monocots that had been estimated to occur between 128–131 mya (ref. 18 ). Gene families Gene families were selected based on prior knowledge about Spirodela biology and on biased representations of gene families, domains and biological processes, identified in our analysis of orthoMCL clusters as well as inter-species comparisons of selected gene families. An outline of our applied pipeline for genome-wide surveys of targeted gene families is shown in Supplementary Fig. 17 . Briefly, we compiled a list of gene identifiers either from publicly available curated gene families or by selection of genes with specific PFAM/InterPro domains from the AHRD annotations [21] (Methods). The Spirodela genome contained very similar patterns of orthologous gene sets in comparison to four representative species (Arabidopsis, tomato, banana and rice), sharing a total of 8,255 common gene families despite a significantly reduced gene number ( Fig. 8 ; Supplementary Fig. 18 ). However, Spirodela clusters generally showed the lowest average gene expansion and copy number, indicating preferred gene losses of duplicated genes in Spirodela or— vice versa —gene retentions in the other species ( Supplementary Table 13 ). A notable exception from the overall conserved gene content was 750 orthoMCL clusters present in all four analysed species except Spirodela. These families included genes involved in water transport by aquaporins, phenylpropanoid, lignin biosynthesis and cell wall organization by expansins ( Supplementary Table 14 ). The loss of these gene families is consistent with the specialized morphology and lifestyle of Spirodela. Overrepresented functional categories of Spirodela-specific genes were enriched for various defence-related processes including antimicrobial peptides and adapted immune responses ( Supplementary Table 15 ) (further details on orthologous gene sets and on gene ontologies under Supplementary Discussion ). Figure 8: OrthoMCL analysis of gene families. The Venn diagram illustrates shared and distinct cluster classes from an orthoMCL analysis of the plant proteomes of Arabidopsis thaliana , Solanum lycopersicum , Spirodela polyrhiza , Musa acuminata and Oryza sativa spp. indica . Non-redundant data sets were used in the analysis. Numbers below each species name show number of all genes in species set and number of clustered genes, respectively. For each division in the Venn diagram, the top line shows the number of orthoMCL clusters and the bottom line the number of total genes in these clusters. The different cluster classes are colour-coded by the number of species containing genes for the respective class. Divisions for each class are shaded according to their abundance in their class with darker shades indicate larger contributions of the particular division. Full size image Morphogenesis and plant body architecture Expansins are cell-wall-loosening proteins [22] involved in many plant processes including cell growth and expansion, root and root hair expansion, fruit softening, ripening and abscission [23] . We analysed α- and β-expansins by an integrative pipeline, which showed reduced copy numbers in Spirodela ( Supplementary Figs 19 and 20 ). Several clades of α-expansin genes were missing in Spirodela including AtEXP 2, 8, 17, 11, 7 and 18. The latter two expansins have been implicated in root hair initiation with AtEXP7 restoring a short root hair phenotype in rice, indicating orthologous functions of this expansin in monocotyledonous species [24] , [25] . Monocotyledonous plants have experienced a great expansion of β-expansins, with 10 detected in banana and on average 20 members in the Poaceae species. However, we detected only three β-expansins in Spirodela, indicating that the expansion continually progressed along the monocotyledonous diversification or a selective decrease of this gene family in Spirodela ( Supplementary Fig. 20 ) (further details on expansins under Supplementary Discussion ). Owing to the high buoyancy of their habitat, aquatic plants like duckweed do not require the vertical structural support like land plants that would be consistent with a reduction of genes involved in cell wall biosynthesis and lignification. Although cell wall biogenesis genes such as CesA, CslA, CslC and CslD were conserved across rice, Arabidopsis and Spirodela ( Supplementary Table 16 ), there were two unique rice clades of CslF and CslH and two unique Arabidopsis clades of CslB and CslG. Spirodela is missing comparable members of CslB, CslE, CslF, CslG and CslH ( Supplementary Fig. 21 ). We found all corresponding GT31 subfamily members in Spirodela, but the total copy number was 46.2% lower than in rice ( Supplementary Fig. 22 ). The missing five clades in the Csl family and the fewer members in the GT31 family are consistent with the low content of 4–16% cellulose in Spirodela [26] in comparison to 62% in rice [27] , which might indicate that the contraction or lack of amplification of the cellulose biosynthesis gene family in Spirodela reflects its reduced requirement for rigid cell walls (further details on cellulose biosynthesis under Supplementary Discussion ). Lignin, a major component of secondary cell wall, plays an important role for support, water transport and stress responses in vascular plants. As shown in previous comprehensive phylogenetic analyses, most lignin biosynthesis gene families experienced rapid and recent duplications; the expansion mainly happened after the speciation between monocotyledonous and dicotyledonous species [28] . Although Spirodela contained nearly the entire lignin biosynthesis gene families with 9 out of 10 families (CAD, CCoAMT, 4CL, CCR, PAL, C4H, COMT, C3H, F5H but not HCT), gene copy number was significantly reduced compared with other monocotyledonous species like sorghum and rice ( Supplementary Table 17 ). This was consistent with previous genome analysis, where gene copy number constituted an important evolutionary force for specialization and traits. In addition to genes catalysing primary lignin biosynthesis, families involved in cell wall crosslinking and lignification also showed reduced copy numbers. We identified only seven members of the laccase multicopper enzymes in Spirodela, for which recent studies had provided experimental evidence for their role in lignification [29] ( Supplementary Fig. 23 ). This was consistent with previous analyses of 3.1% lignin in Spirodela [30] in comparison with 18% in rice straw [27] (further details on lignin biosynthesis and laccases under Supplementary Discussion ). Ecological adaptation Spirodela polyrhiza can undergo an environmentally induced developmental switch from protein-rich vegetative leaf-like ‘fronds’ to a starch-rich dormant stage called ‘turion’ [31] . Unlike the linked vegetative fronds via stipule, turions fall from the mother fronds once mature after starch accumulation. They sink to the bottom of a pond and germinate into new fronds by using starch as energy. These functions require genes for starch biosynthesis including AGPase, SS plus GBSS, BE and DBE. Spirodela contained very similar gene family compositions as Arabidopsis ( Supplementary Table 18 ). The conservation of starch gene families from phylogenetic analysis for Spirodela, rice, maize and Arabidopsis argues for their essential functions. The clades of AGPase large subunit and DBE had multiple members, whereas all others contained only one single member for the corresponding subgroup. SpBEIII did not cluster with any clade, but provided a separate branch as a Spirodela-specific BE member, suggesting that it might have evolved into a special function from their common ancestor ( Supplementary Fig. 24 ) (further details on starch biosynthesis under Supplementary Discussion ). The high growth rates of Spirodela require the efficient usage of nutrients. Nitrogen is generally a major limiting factor of plant growth and a primary component in fertilizers to promote crop growth. However, leaching of fertilizers, increasing amounts of sewage and wastewater from a steadily growing world population results in water pollution. Spirodela has been successfully exploited for wastewater remediation because of its ability to remove nitrogen with high efficiency, particularly in the form of ammonia, from polluted water [5] . Glutamine synthetase (GS) and glutamate synthase (GOGAT) are the core enzymes of the GS/GOGAT cycle in plants, the major biochemical module for ammonium assimilation. Despite a genome-wide reduction in gene number, copy numbers of these enzymes were retained or even amplified in Spirodela with up to four times more copies of Fd-GOGAT in Spirodela compared with Arabidopsis and rice ( Fig. 9 ; Supplementary Fig. 25 ) (further details on nitrogen efficiency under Supplementary Discussion ). Figure 9: Spirodela characteristic pathways. ( a ) A schematic diagram of nitrogen assimilation in higher plants is illustrated. Spirodela shows a high overrepresentation of enzymes of the GS/GOGAT cycle, the major module for ammonia assimilation and consistent with the high ability of Spirodela to remove ammonia from sewage and wastewaters. Copy numbers for each gene are shown in red for Spirodela, blue for rice and green for Arabidopsis. ( b ) A highly simplified scheme of the regulatory network of the juvenile-to-adult phase transition in Arabidopsis is illustrated. Most genes have several, functionally similar paralogs and are only shown for simplicity reasons by one gene symbol. For example, APETALA1, CAULIFLOWER and FRUITFUL are close paralogs promoting the onset of an inflorescence meristem but are represented only by one gene symbol, AP1. Gene groups having either similar copy numbers or being overrepresented in Spirodela are shown in red; those that have significantly reduced numbers are shown in blue. Full size image Development and reproduction Flowering plants undergo a series of distinct phase transitions during their life cycle, including the progression from a vegetative or juvenile phase to an adult phase with competency for sexual reproduction (flowering). Neoteny, the prolongation of juvenile traits, is a common phenomenon in the evolution of plant organs. The frond of the Lemnoideae has been characterized as embryonic or juvenile tissue, or as a cotyledon-like plant, iteratively bearing new cotyledons ( Supplementary Fig. 1 ). Although Spirodela has an increased copy number of repressors of the transition from juvenile to adult phase in comparison to Arabidopsis and rice, components of the regulatory network enhancing the progression through the adult phase and the onset of an inflorescence meristem were reduced ( Fig. 9 ; Supplementary Table 19 ), for example, SPB ( Supplementary Fig. 26 ), MADS-box ( Supplementary Fig. 27 ) and PEBP gene families ( Supplementary Fig. 28 ). In Arabidopsis, the microRNA of miR156 is necessary and sufficient to promote the juvenile phase and inhibit the transition to the adult growth [32] . Copies of miR156 were highly abundant in Spirodela, with 24 loci, or up to 32 loci if highly similar isoforms were included, consistent with the pattern of preferentially retained repressors of the adult phase, whereas Arabidopsis had only 10 and rice had 19 loci. The opposite was true for miRNA169, involved in drought tolerance [33] , and miRNA172, involved in the switch from juvenile to adult phase [34] , which were reduced from 9 and 5 copies found in Arabidopsis and tomato, respectively, to 1 ( Supplementary Table 9 ) (further details on the transition from juvenile to adult phase under Supplementary Discussion ). In higher plants, gene number and genome size seem to be not correlated. Although Arabidopsis thaliana has a genome size similar to Spirodela, it contains ~28% more genes. The low gene count of Spirodela could in part be due to the structural reduction and juvenile nature reducing the need for and consequently the retention or duplication of genes acting in the adult phase. In addition, Spirodela differs from previously reported angiosperm genomes in its lack of recent WGDs and retrotranspositions. The lower gene number in Spirodela may therefore be simply a consequence of the ongoing non-functionalization and loss of one copy of a duplicated gene pair, a major fate of gene duplication [19] . We propose that the predominant vegetative reproduction and low flowering frequency as well as the reduced and simple plant body of Spirodela is at least in part a consequence of the re-engineering of the genetic network that controls transitions to the adult and flowering growth phases. Interestingly, structural reduction increases in the Lemnoideae from the more ancient species like Spirodela towards the more derived members such as Wolffia ( Fig. 1 ). Genomes of duckweeds should therefore present an excellent opportunity to study how different degrees of neoteny translate into molecular changes of developmental networks and gene families. As Spirodela provides us with a unique and fascinating biology, its genome sequence will serve us for future evolutionary and comparative genomic studies among angiosperms. In addition to basic question in plant evolution and development, applications of duckweeds in water remediation and as a renewable energy source can now be further optimized. The genome sequence of Spirodela provides the first step to identify, understand and improve relevant traits for specific target applications. Genomic DNA isolation One cluster of 3–5 fronds of Spirodela polyrhiza strain 7,498, which were clonally grown from one plant to reduce potential sequence polymorphism, was aseptically transplanted into half-strength Schenk and Hildebrandt basal salt mixture (Sigma, S6765) with 1% sucrose liquid medium at pH 5.8. The cultures were kept in a growth-chamber, maintained at 100 μmol m −2 s −1 and 23 °C through a 16 h-light, 8 h-dark photoperiod [31] . High molecular weight of nuclear DNA was extracted by adaption of a nuclei isolation procedure and the CTAB method [35] . Simply, after grinding 10 g of frozen tissue in liquid nitrogen, nuclei were isolated with a sucrose-based buffer, and then suspended in 50 ml CTAB extraction buffer. The isolated DNA was digested with 50 μg ml −1 RNase for 1 hour at 37 °C. The quality and quantity were checked with a 1% gel and measured with Nanodrop 1000. Haploid genome size estimation For flow cytometric genome size estimations 10 mg of fresh duckweed tissue were chopped together with similar amounts of an internal reference standard Raphanus sativus ‘Voran’ (IPK gene bank accession number RA 34, 543 Mb) with new razor blades in propidium iodide-containing nuclei isolation buffer [36] . Measurements were performed on a FACStarPLUS cell sorter (BD Biosciences, San Jose, CA, USA). The calculated average value is based on at least 10 independent measurements performed on separate days. Genome sequencing and sequence assembly A high-quality genome sequence was produced with the Roche/454 and Sanger ABI-3730XL platforms, using the whole-genome shotgun sequencing method [37] , [38] . Sequencing reads for the nuclear genome were collected with the Roche 454 XLR next-generation sequencing platform at the Department of Energy Joint Genome Institute (JGI) in Walnut Creek, CA, USA, according to the manufacturer’s specification (454 Life Sciences, Branford, CT, USA). Two linear Roche 454 libraries (8 runs, 2.95 Gb) and one 5.7 kb insert size paired library (343.4 Mb) were sequenced with standard XLR protocols. Paired ends were also generated from BAC and fosmid libaries and 24 entire finished fosmids were obtained using standard protocols on ABI3730XL machines at the HudsonAlpha Institute in Huntsville, AL, USA, and the JGI according to the manufacturer’s specification (Life Technologies, Grand Island, NY, USA). The assembly was generated using Newbler version 2.6 with default parameters after trimming poor bases from ends and masking vector sequences. Physical map and pseudomolecules A Spirodela BAC library was constructed from high-molecular weight nuclear DNA [35] . The DNA was partially digested with HindIII, double size-selected and ligated into pIndigoBAC-5 (HindIII-cloning Ready, Epicentre, BACH095H, Madison, WI, USA). A total of 15,360 Spirodela BAC clones with an average insert size of 110 kb representing 10 × genome equivalents were fingerprinted with the SNaPshot HICF fingerprinting method using the LIZ1200 size standard as described somewhere else [39] . Of the 15,360 fingerprinted clones, 11,770 clones (76.6%) were suitable for contig assembly. There was on average one restriction fragment every 1.19 kb. The final FPC map spanned 200 Mb and contained 269 singletons and 11,501 BAC clones, which were integrated into 320 contigs. In the physical map, 23 contigs had more than 100 clones each, 62 contigs had 50–99 clones each, 160 contigs had 10–49 clones and the residual 75 had <10 clones. Based on the physical map integration, the Newbler scaffolds were ordered by the FPC draft sequence function and pseudomolecules were constructed from joined scaffolds. Scaffolds within one pseudomolecule were interlaced by a stretch of 500 undefined bases (‘N’s). Cytogenetics To align the 32 BAC-based pseudomolecules with linkage groups represented by individual chromosome pairs, we applied FISH. BACs with a low repeat content according to RepeatMasker ( http://www.repeatmasker.org/ ) analysis were assembled into contigs spanning the physical map of Spirodela polyrhiza . These BAC contigs were subdivided into appropriate probes for FISH. Metaphase chromosome spreads of Spirodela were prepared from young root tips treated with 0.002 M 8-hydroxyquinoline for 1 h on ice before fixation in absolute ethanol: acetic acid (3:1, v / v ) for 48 h and digestion for 90 min at 37 °C in 1% cellulase and 1% pectinase in 0.01 M sodium citrate at pH 4.8. Digested root tips were squashed in 75% acetic acid on slides and frozen on dry ice. BAC probe labelling, FISH, microscopic evaluation and image processing were performed as described [40] . Assembly check The so called ‘assembly checker’ is based on sequence content assessment by masking one sequence set with another via the programme vmatch ( http://www.vmatch.de ). The approach introduces a versatile alternative method for the quantification of assembly completeness. Whole-genome sequence sets, like transcripts, reads and BESs are used as test sets to determine their percent base-pair coverage with the genome assembly. After the evaluation of different matching stringency, the parameters setting ‘−l 50 −e 1’ (=minimum hit length 50 bp, maximal 1 mismatch or indel per 50 bp) was found to be suitable for the Spirodela sequence sets. Here the matching of two different random sets of 1 × genome coverage against each other gave 63% coverage, which is exactly the Lander–Waterman expectation. RNA isolation and cDNA sequencing To collect a diverse set of expressed genes, Spirodela polyrhiza was grown under different light–dark cycles (24 h/0 h, 16 h/8 h, 12 h/12 h, 8 h/16 h and 0 h/24 h) and collected at time points that represent various states of the circadian clock (02:00, 06:00, 10:00, 14:00, 18:00 and 22:00). In addition, Spirodela polyrhiza cultures were treated by various stress conditions (heat treatment at 37 °C, cold treatment at 0 °C, desiccation on agar plate, high pH value of 9, UV exposure, 20 mg l −1 CuCl 2 , 300 mg l −1 KNO 3 , 250 nM ABA, 10 μM kinetin, 300 mM mannitol) and samples were collected at different exposure times (0.5 h, 1 h, 3 h, 6 h, 12 h and 24 h). Fresh tissue (0.2 g) was collected from each conditions and flash-frozen in liquid nitrogen. High-quality total RNA was extracted with the RNeasy Plant Mini Kit (Qiagen, 74904). The on-column DNase I was used to remove contaminating genomic DNA (Qiagen, 79254). We used gel electrophoresis and Nanodrop 1,000 to assess RNA quality and quantity. Finally, equal amounts of RNA were pooled from each sample. The library was constructed for RNA samples and sequenced with the ‘454’ platform. ESTs were assembled using the Joint Genome Institute EST sequence-processing pipeline. Briefly, raw 454 EST sequences were trimmed for vector and adaptor/linker sequences and poor reads. Contaminants were also screened and filtered by BLAST alignment. ESTs were clustered using malign and assembled using CAP3 to build tentative consensus sequences. Repeat analysis Kmer frequencies are a repeat library independent and thus unbiased method to access the repetitive portion of a genome. The programme tallmyer [41] from the programme suite genome tools ( http://genometools.org/ ) was used to calculate the frequency of each 16-mer in the respective genome assemblies and other sequence sets. Complete LTR retrotransposons where identified in a de novo approach with the programme LTR-STRUC [42] . Quality filtering was based on <30% tandem repeat content, at least one typical inner protein domain, manual dot plot inspection and removal of overlapping sequences. Additional complete LTR-retrotransposons were detected by homology search against the full-length sequences. The insertion age of full-length LTR-retrotransposons was derived from the divergence (emboss distmat with Kimura 2 parameter distance) between the left and right LTR sequences, which were identical after transposition as described elsewhere [43] . Transposons and rRNA genes were annotated by the wublast version of RepeatMasker-open-3-3-0 ( http://www.repeatmasker.org ) against the mipsREdat (REdat_v9.3, 387 Mb, 56,169 entries). The RepeatMasker output was subjected to two post-processing filter steps, removal of low confidence hits (length <50 bp or score <250 or identity <60%) and purification of overlapping annotations in a priority-based approach, where higher score hits were assigned first and overlapping lower score hits either shortened or, if the overlap exceeded 90% of their length, removed. Tandem repeat sequences were detected with the programme Tandem Repeats Finder [44] under default parameters. Classification of the tandem repeats were based on their monomer length and divided into microsatellites (2–9 bp), minisatellites (10–99) and satellites (≥100bp). Overlapping annotations were joined and classified as hybrid type, if they contained more than one of the three classes. Gene prediction and annotation Gene models were derived from consensus gene predictions based on de novo gene finders, transcript data and protein homologies. EST assemblies of Spirodela and of two sea grasses, Posidonia oceanica and Zostera marina [45] , were used as transcript evidences. Heterologous protein evidence was based on protein sequences of four monocotyledonous species—Brachypodium, maize, sorghum and rice—and three dicotyledonous species, Arabidopsis, poplar and Vitis. For evidence by homology, spliced alignments were generated by GenomeThreader [46] using an initial seed size of seven amino acids for protein and 16 bp for nucleotide alignments. For de novo gene finders, a training set was derived from mapping the Spirodela EST assemblies and high-quality protein families to scaffold sequences. As high-quality proteins, we selected orthologous gene families from the PLAZA database [47] , for which at least five distinct plant species had members differing by a maximum of 2% in the protein sizes from the mean family sequence size. Next, we performed multiple sequence alignments of the selected families applying MUSCLE [48] to confirm sequence similarity and size consistency in the alignments. Spliced alignments to Spirodela genomic scaffolds were computed using GenomeThreader and filtered for full-length alignments including start and stop codons, high similarity (blosum62 score ≥ twice size of alignment) and size consistency with the respective gene family. Remaining gene models for training were selected to be non-redundant both in terms of individual, overlapping mappings of members of one family as well as mappings of one family to multiple genomic locations. To derive full-length Spirodela transcripts from the EST assemblies, candidate ORFs were predicted by applying ORFpredictor [49] with pre-computed tblastx comparisons against a database compilation of Arabidopsis, Sorghum and Brachypodium proteins. Only ORFs with similarity to known proteins and full-length alignments to a genomic position of Spirodela scaffolds including start and stop codon were retained. Finally, we compiled a non-redundant training set as described above for the PLAZA proteins. Using the non-redundant data sets described above, we trained four de novo gene prediction tools, Augustus, Snap, GlimmerHMM and GeneID [50] , [51] , [52] , [53] and determined genome-wide predictions using the Spirodela-specific parameter sets of each tool. An additional gene finder, Fgenesh+, was run using a monocotyledonous-specific parameter matrix [54] . Next, the statistical combiner Jigsaw was trained using our training set, mapped homologies and gene models predicted by our set of de novo gene finders [55] . The resulting gene models constituted version 1.0. For historical reasons, an independent set of predictions was made with a new self-training ab initio gene finder, GeneMark-ES-GC, developed for compositionally heterogeneous genomes (Lomsadze and Borodovsky, unpublished). The GeneMark-ES-GC gene predictions were later merged with the models produced by computational homologies and models the other de novo predictions including the Jigsaw models. Upon merging, de novo models with no significant homology (blastp E -value >10–10 versus UniprotKB/Swissprot) were included, if at least two independent predictions supported an identical gene structure. Finally, models from the training set were integrated into this set of gene models to obtain the final set of consensus gene predictions, to which we refer as version 2.0. Mature miRNA sequences of all plant species present in miRBase version 19 (ref. 56 ) were mapped to the Spirodela whole-genome assembly using vmatch [57] , allowing up to two mismatches. Subsequently, 150-bp flanking sequences adjacent to the 5′- and 3′-boundaries of putative miRNAs were retrieved and their secondary structure was predicted using RNAfold [58] with standard settings. The structure was evaluated using MIRcheck with default settings [59] . Putative miRNAs passing MIRcheck were retained and overlapping loci of matched miRNAs were concatenated and annotated as one miRNA. Tandem genes An undirected graph was constructed from a self-comparison of each proteome using blastp with protein identifiers as nodes and edges, which specified similarity matched between two proteins and were weighted by expectation values. A first filter removed all matches above a threshold E -value E >10–10. Next, only edges connecting two proteins with a genomic distance of <10 dissimilar intervening genes were retained. Tandem clusters were determined as connected components from this trimmed graph. Organellar insertions The assembled nuclear genome of Spirodela was compared by blastn against the Spirodela plastid genome (JN160603) [35] and the mitochondrial genome (JQ804980) [60] , respectively, to identify the insertion of organellar sequences into the nuclear genome. We retained all hits longer than 50 bp and hits were categorized by their size. Heat maps Heat maps and stacked bar charts are used to visualize and compare specific chromosomal content from a bird’s eye perspective. The higher-level heat map data were created by sliding along the chromosome with a 0.1-Mb window size and 0.02-Mb shift length and determining for each window the number and percentage of bp coverage of the respective element type, like genes or LTR-retrotransposons. For kmer frequencies the mean and median values per window was used. The density values were corrected for the number of Ns per window, if the N content exceeded 60% the value was set to null and drawn in grey colour. The number value was extrapolated to number per Mb to facilitate comparisons. The heat maps were created from the obtained density values using the python pylab module in combination with the jet colour map (low to high values from blue to red). A more detailed insight into the annotation structure was achieved with the integrative genome viewer ( http://www.broadinstitute.org/igv/ ) by defining customized tracks for the different element types and kmer values in combination with special colour codes and display options. Synteny Analysis of genome duplications were based on all-against-all blastp comparisons between non-redundant gene sets of the respective species ( E -value cutoff E <10–10). Intra- and intergenomic duplicated segments were identified by a combination of quota alignments [20] (exploring various quota settings for the expected evolutionary history of genome duplications) and manual inspection and curation of dot plots. Genes between candidate duplications were aligned by a global alignment similar to the methods described elsewhere [61] . Statistical significance of candidate duplications was evaluated by a Monte Carlo test. Briefly, the gene order in one genome was randomly shuffled 1,000 times by exchanging gene identifiers, and gene alignments were recomputed according to the initial genomic borders of candidate segments. Alignments of the random genomes were ranked by the number of aligned homologues and all candidate duplications with a P -value <0.001 were retained. Synonymous Ks and non-synonymous Ka substitution rates for duplicated genes were determined with Smith–Waterman alignments of protein sequences and subsequently derived codon-based alignments [62] . Rates were computed by the Nei–Gojobori method as implemented in the KaKsCalculator tool [63] . Previous studies had shown a strong dependency of Ks values on the GC3 composition of gene pairs [20] , [64] . We therefore analysed Ks values of gene pairs separately for GC3-high (GC3>75% for both genes), -medium (exactly one gene with GC3>75%) and -low (GC3≤75% for both genes) pairs. Divergence time estimates were based on histogram peak Ks values of the low pairs and a molecular clock of λ =6.5 × 10–9 synonymous substitutions per site and year [65] . Divergence times T were computed as T =2 λ Ks. We emphasize, however, that all estimates might be biased by the unusual GC3 content of Spirodela genes and possible rate differences that had been reported in monocots [65] . Gene family list To extend the strict gene family list and include closely related candidate in-paralogues from distinct clusters, we determined for each cluster the minimal intra-cluster similarity/threshold T of its members using an all-against-all blastp comparison between all genomes. The minimal intra-cluster threshold Ti was defined as the minimal expectation value E of all pairwise similarity comparisons between members of cluster i. In addition, it was restricted to a maximal value of E ≤10–30. Next, we expanded our strict gene family list by including all matches that exceeded threshold Ti to any member of the ith cluster and derived by this procedure the extended gene family list. For both gene lists, multiple protein sequence alignments were computed using MUSCLE [48] . Alignments were checked by Gblocks [66] and manual curation. Phylogenetic trees were constructed using FastTree [67] . Visualization and analysis of phylogenetic trees was performed with custom-made python scripts, the python module ETE2 and iHOP [68] , [69] . Trees were manually inspected for reduced and amplified copy numbers of orthologous genes between Spirodela and other plant species and results were analysed by searches of the known literature. Accession numbers: The genome sequence of Spirodela polyrhiza strain 7498 has been deposited in DDBJ/EMBL/GenBank nucleotide core database under accession code ATDW00000000 . BAC End sequences have been deposited in the GenBank GSS database under accession codes JY978532 to KG007076 . Fosmid sequences have been deposited in the GenBank nucleotide core database under accession codes AC254537 to AC254559 How to cite this article: Wang, W. et al. The Spirodela polyrhiza genome reveals insights into its neotenous reduction fast growth and aquatic lifestyle. Nat. Commun. 5:3311 doi: 10.1038/ncomms4311 (2014).